Requirement of calcium-activated chloride channels in the activation of mouse vomeronasal neurons In terrestrial vertebrates, the vomeronasal organ (VNO) detects and transduces pheromone signals. VNO activation is thought to be mediated by the transient receptor potential C2 (TRPC2) channel. The aberrant behavioural phenotypes observed in TRPC2−/− mice are generally attributed to the lost VNO function. Recently, calcium-activated chloride channels have been shown to contribute to VNO activation. Here we show that CACCs can be activated in VNO slice preparations from the TRPC2−/− mice and this activation is blocked by pharmacological agents that inhibit intracellular Ca 2+ release. Urine-evoked Cl − current is sufficient to drive spiking changes in VNO neurons from both wild-type (WT) and TRPC2−/− mice. Moreover, blocking Cl − conductance essentially abolishes VNO activation in WT neurons. These results suggest a TRPC2-independent signalling pathway in the VNO and the requirement of calcium-activated chloride channels currents to mediate pheromone activation. Our data further suggest that TRPC2−/− mice retain partial VNO function. In terrestrial vertebrates, the vomeronasal organ (VNO) detects and transduces pheromone stimuli using a set of signalling molecules distinct from those used in the main olfactory epithelium (MOE). The mammalian VNO expresses three distinct families of G-protein-coupled receptors, V1Rs, V2Rs and FPRs [1] , [2] , [3] , [4] , [5] , [6] , [7] . On binding to their ligands, these receptors initiate signalling cascades that activate phospholipase C to elevate the levels of inositol 1,4,5-trisphosphate (IP3), diacylglycerol and their metabolites [8] , [9] , [10] , [11] , [12] , [13] , [14] . These events are thought to lead to the activation of the non-selective cation channel TRPC2, a member of the TRP superfamily of non-selective ion channels [15] , [16] , [17] . TRPC2 is highly expressed in the VNO neurons and is enriched in the sensory microvilli of the dendrites [15] , [16] , [17] , [18] . Genetic removal of the TRPC2 channel from the mouse genome results in a significant loss of pheromone-triggered responses in VNO neurons and aberrant innate behaviours [19] , [20] , [21] . However, pheromone-triggered responses are still detected from the VNO of TRPC2−/− mice [20] , [22] , [23] . Studies have suggested TRPC2-independent signalling in the VNO, but the ionic mechanism is unclear [22] , [23] . In a recent study, calcium-activated chloride channel (CACCs) were found to be activated by urine in the mouse VNO [24] . Although it is assumed that CACC currents act downstream of TRPC2 to amplify its activation, there is no experimental evidence to distinguish whether the two signalling pathways act sequentially or independently. In this study, we find that the Cl − conductance contributes a significant portion to the urine-evoked current in VNO slice preparation. We show that activation of this conductance is triggered by both Ca 2+ entry through the TRPC2 channel and Ca 2+ release from intracellular stores. In the absence of TRPC2, the activation of the Cl − conductance is sufficient to trigger spiking activity in the VNO neurons. On the other hand, blocking Cl − conductance greatly reduces VNO activation in both wild-type (WT) and TRPC2−/− neurons. Our results suggest a TRPC2-independent signalling pathway in the VNO neurons and the requirement of CACC currents to mediate pheromone activation. Urine-evoked responses in slice preparations of VNO The sensory neurons in the VNO form a pseudostratified sheet in which the dendrites of the neurons are exposed to the apical lumen and the cell bodies are insulated by the sustentacular cells [25] . Only a handful of studies have investigated pheromone-induced responses in VNO neurons in this native configuration [9] , [26] , [27] , [28] . We therefore performed patch clamp experiments in slice preparations of the VNO to assess the contributions of different signalling mechanisms to VNO responses. We used mouse urine as the pheromone source to activate VNO neurons. Previous studies showed that urine only activated a fraction of the neurons and elicited a range of responses [28] , [29] , [30] . This is likely because of the fact that each VNO neuron expresses a single type of vomeronasal receptor [1] , [2] , [3] , [4] , [5] , [6] , [7] and the responses are highly specific [26] . To accurately assess the responses, we analysed all the cells recorded in VNO slices and plotted the current amplitude histogram ( Fig. 1a–c ). It was apparent that under control conditions, the responding cells showed amplitudes that were significantly larger than 2× random noise of the filtered records (0.2 pA). We thus only analysed responses with amplitude larger than 0.4 pA. Approximately 40% of the cells showed reliable responses to repeated urine stimulation (12 out of 29 cells, 41.4%). The percentage of responsive cells was consistent with previous findings using Ca 2+ imaging to study urine-evoked responses in the same preparation [29] , [30] . 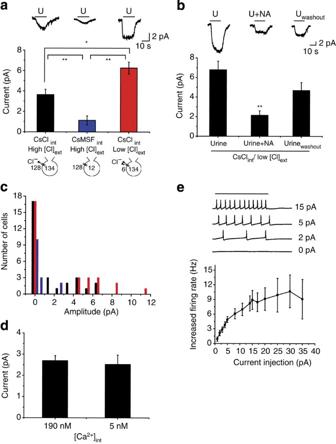Figure 1: Contribution of Cl−conductance to urine-evoked current in the VNO. (a) Urine-evoked whole-cell currents recorded in WT mice with CsCl (left and black bar;n=12), CsMSF (middle and blue bar;n=5) internal solutions or gluconate-substituted external solution (right and red bar;n=12). Top, sample traces of the recordings. Black lines above the traces indicate the duration of urine application. Middle, average response amplitude of inward currents. Bottom, illustration of intracellular and extracellular Cl−concentrations. (b) Sample traces and bar graph showing the effects of niflumic acid on urine-evoked currents. Response currents are recorded under control, niflumic acid (NA) treatment and after washout (Uwashout). Traces shown are from the same cell. Seven cells were recorded, with one cell lost during washout. (c) Response amplitude histogram for the currents shown ina, with 0.5 pA bin size. Black, blue and red bars indicate the recording conditions illustrated ina. (d) Response amplitudes at intracellular Ca2+concentrations of 190 nM (n=6) and 5 nM (n=7). (e) Increase in spiking rates as a function of depolarizing current injection. Top, sample traces of spike patterns in 0, 2, 5 and 15 pA injection. Bar above the traces indicates duration of current injection. Error bars indicate standard errors. Bottom, summary of the current injection experiment (n=6). *P<0.05 and **P<0.01 (pairwiset-test). All pairs marked with * havepost hocanalysis of variance test,P<0.01. ext, external; int, internal. Figure 1: Contribution of Cl − conductance to urine-evoked current in the VNO. ( a ) Urine-evoked whole-cell currents recorded in WT mice with CsCl (left and black bar; n =12), CsMSF (middle and blue bar; n =5) internal solutions or gluconate-substituted external solution (right and red bar; n =12). Top, sample traces of the recordings. Black lines above the traces indicate the duration of urine application. Middle, average response amplitude of inward currents. Bottom, illustration of intracellular and extracellular Cl − concentrations. ( b ) Sample traces and bar graph showing the effects of niflumic acid on urine-evoked currents. Response currents are recorded under control, niflumic acid (NA) treatment and after washout (U washout ). Traces shown are from the same cell. Seven cells were recorded, with one cell lost during washout. ( c ) Response amplitude histogram for the currents shown in a , with 0.5 pA bin size. Black, blue and red bars indicate the recording conditions illustrated in a . ( d ) Response amplitudes at intracellular Ca 2+ concentrations of 190 nM ( n =6) and 5 nM ( n =7). ( e ) Increase in spiking rates as a function of depolarizing current injection. Top, sample traces of spike patterns in 0, 2, 5 and 15 pA injection. Bar above the traces indicates duration of current injection. Error bars indicate standard errors. Bottom, summary of the current injection experiment ( n =6). * P <0.05 and ** P <0.01 (pairwise t -test). All pairs marked with * have post hoc analysis of variance test, P <0.01. ext, external; int, internal. Full size image Urine activates a Cl − conductance We specifically examined the contribution of the CACCs to urine-induced currents ( Fig. 1a,b ). We performed whole-cell recordings using intracellular solutions with Cl − substituted by the non-permeable anion methanesulfonate (MSF − ). Under this condition, we set the reversal potential for Cl − to −60 mV so that there was no net flow of Cl − across the membrane. Substitution of intracellular Cl − with MSF − resulted in a reduction of ∼ 70% of urine-induced inward current (from 3.65±0.50 to 1.12±0.45 pA; Fig. 1a ). Conversely, substitution of extracellular Cl − with non-permeable gluconate without altering intracellular Cl − led to an increase in the amplitude of the inward current (from 3.65±0.50 to 6.25±0.59 pA; Fig. 1a ). Furthermore, treatment of niflumic acid, a Cl − channel blocker, reduced urine-evoked currents by ∼ 70% (from 6.77±0.89 to 2.13±0.46 pA; Fig. 1b ), similar to the effect of replacing intracellular Cl − . These findings demonstrated the presence of a Cl − current in urine-evoked response in VNO neurons. Sensitivity to small currents in VNO neurons In agreement with a previous study [27] , the currents recorded from the vomeronasal neurons in slices were within picoampere range. To test whether the small currents were caused by rapid run-down as a result of low Ca 2+ concentration in the pipette, we used intracellular solutions containing either 5 mM EGTA/2 mM Ca 2+ or 1 mM EGTA/0 mM Ca 2+ . The Ca 2+ concentrations in the pipette solutions were estimated to be 190 and 5.55 nM, respectively [31] . We found little difference in the responses under these two conditions ( Fig. 1d ). Overall, urine application induced inward currents of 2–12 pA when the cells were voltage clamped at −60 mV ( Fig. 1c ). These currents were significantly smaller than those reported for olfactory neurons, in which odour-evoked currents were 10–100 times larger [32] , [33] . We reasoned that the small current was characteristic of the VNO neurons based on the fact that field potential recordings of urine-evoked responses in VNO epithelia ( ∼ 100–200 μV) were about 100 times smaller than those of odour-evoked potential from the olfactory epithelia (10–20 mV) under similar recording conditions [29] , [32] . To further test whether this small current was physiologically relevant, we examined the relationship between input current and the spiking activities of the VNO neurons. Under current clamp condition, current injection as low as 1 pA was able to change spiking frequency of the VNO neurons ( Fig. 1e ). The change in spiking rate was most sensitive in the range of 1–5 pA injection and reached a plateau at 15 pA ( Fig. 1e ). The sensitivity to small current was consistent with that observed in dissociated cells [34] and was likely the result of the large input resistance (1–3 GΩ) of the VNO neurons [9] , [34] . Urine-activated Cl − current requires Ca 2+ We next tested whether extracellular and intracellular Ca 2+ concentration changes affected urine-induced responses. In these experiments, we substituted Na + with Li + in both bath and intracellular solutions to prevent possible membrane currents operated by the Na + /Ca 2+ exchanger in response to changes of intracellular Ca 2+ level [35] , [36] . When extracellular Ca 2+ concentration was reduced from 2 mM to 1 and 0 mM, we observed corresponding decreases in urine-evoked currents (from 4.12±0.56 pA to 2.71±0.32 and 1.65±0.31 pA, respectively; Fig. 2a,b ). This experiment suggested that Ca 2+ was required for urine-evoked currents. 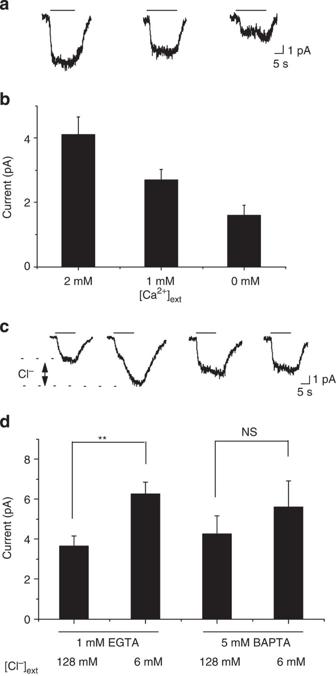Figure 2: Urine-activated Cl−current requires Ca2+. Sample traces (a) and average amplitude (b) of whole-cell currents in response to urine activation recorded under the three different extracellular Ca2+concentrations ([Ca2+]ext). Sample traces (c) and average amplitude (d) of whole-cell currents recorded using 1mM EGTA (n=12) or 5 mM BAPTA (n=6) in pipette solution at different extracellular Cl−concentrations ([Cl]ext). The same cells were recorded before and after external Cl−substitution with gluconate. The difference in current amplitude indicated incis attributed to Cl−channels. Black lines above the traces indicate the duration of urine application. Error bars indicate standard errors. **P<0.01; NS, not significant. Figure 2: Urine-activated Cl − current requires Ca 2+ . Sample traces ( a ) and average amplitude ( b ) of whole-cell currents in response to urine activation recorded under the three different extracellular Ca 2+ concentrations ([Ca 2+ ] ext ). Sample traces ( c ) and average amplitude ( d ) of whole-cell currents recorded using 1mM EGTA ( n =12) or 5 mM BAPTA ( n =6) in pipette solution at different extracellular Cl − concentrations ([Cl] ext ). The same cells were recorded before and after external Cl − substitution with gluconate. The difference in current amplitude indicated in c is attributed to Cl − channels. Black lines above the traces indicate the duration of urine application. Error bars indicate standard errors. ** P <0.01; NS, not significant. Full size image We next examined the requirement of intracellular Ca 2+ in activating the CACC currents. We manipulated intracellular Ca 2+ concentrations using two Ca 2+ chelating agents, EGTA and BAPTA, in the intracellular solutions. BAPTA had been shown to have a faster dynamics in chelating Ca 2+ than EGTA and was expected to be more effective in suppressing the increase in intracellular Ca 2+ (ref. 37 ). We thus used intracellular solutions containing 1 mM EGTA/0 mM Ca 2+ and 5 mM BAPTA/0 mM Ca 2+ , with the estimated Ca 2+ concentrations to be 5.55 and 0.87 nM, respectively [31] . In cells recorded with 1 mM EGTA, substitution of external Cl − ions with non-permeable anions increased urine-evoked currents by 71% (from 3.65±0.46 to 6.25±0.59 pA; Fig. 2c,d ). In contrast, currents recorded using intracellular solution with 5 mM BAPTA were less sensitive to external Cl − substitution, increased by 31% (from 4.25±0.90 to 5.6±1.30 pA; Fig. 2c,d ). The basal current recorded with 5 mM BAPTA in pipette solution was slightly higher than those recorded with 1 mM EGTA internal solution (4.25±0.90 versus 3.65±0.50 pA; Fig. 2c,d ). This effect might have resulted from reduced activation of calcium-activated potassium channels in the VNO neurons recorded with high intracellular BAPTA [38] , [39] . Nevertheless, maintaining low intracellular Ca 2+ levels significantly reduced the Cl − component of urine-activated response. Activation of Cl − current in TRPC2−/− VNO neurons We then tested whether CACCs could be activated in the absence of TRPC2 channel. We recorded urine-evoked currents in VNO neurons from TRPC2−/− mice [20] and found that the currents were reduced by ∼ 50% when compared with those from WT mice (1.88±0.34 versus 3.65±0.50 pA; compare Figs 1a with 3a ). We further analysed the contribution of Cl − current in TRPC2−/− neurons. Strikingly, we observed that the urine-evoked inward currents were reduced to near zero (−0.05±0.69 pA) when intracellular Cl − was substituted with MSF − . This finding suggested that the inward current was carried entirely by the Cl − conductance in TRPC2−/− neurons ( Fig. 3a ). Conversely, reducing extracellular Cl − to 6 mM increased urine response significantly (5.66±1.02 pA; Fig. 3a ). We parsed out the contribution of Cl − versus non-Cl − current to urine-evoked response in WT and TRPC2−/− VNO ( Fig. 3b ). In WT mice, altering external Cl − concentration only affected the Cl − current but not the non-Cl − components. In TRPC2−/− background, the non-Cl − current was eliminated, but the Cl − currents was only marginally reduced (2.43pA, WT; 1.93 pA, TRPC2−/−). Thus, ∼ 80% of the urine-evoked inward current carried by Cl − was retained in TRPC2−/− mutants. This finding suggested mainly a TRPC2-independent mechanism for CACC activation. 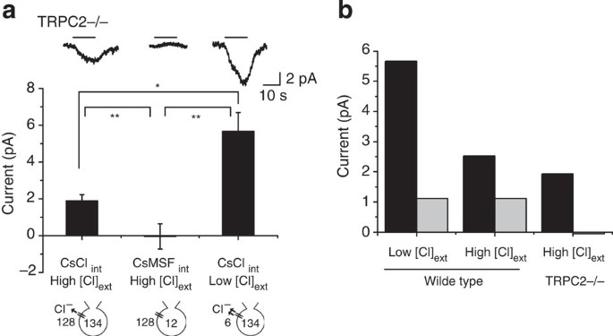Figure 3: CACC activation is independent of TRPC2. (a) Traces and bar graph of urine-evoked whole-cell current recorded in TRPC2−/− mice with CsCl (left;n=7) and CsMSF (middle;n=5) internal solutions and gluconate-substituted external solution (right;n=5). Bars show the average response amplitude of inward currents. (b) Contribution of Cl−and non-Cl−conductance to urine-evoked currents in WT and TRPC2−/− mice. Current amplitude attributed to Cl−component (black bars) was calculated by subtracting the amplitude recorded using CsMSF from that using CsCl internal solution for both the WT and the TRPC2−/− VNO. The non-Cl−component (grey bars) was the current recorded using CsMSF internal solution. *P<0.05 and **P<0.01 (pairwiset-test). All pairs marked with * havepost hocanalysis of variance test,P<0.01. ext, external; int, internal. Figure 3: CACC activation is independent of TRPC2. ( a ) Traces and bar graph of urine-evoked whole-cell current recorded in TRPC2−/− mice with CsCl (left; n =7) and CsMSF (middle; n =5) internal solutions and gluconate-substituted external solution (right; n =5). Bars show the average response amplitude of inward currents. ( b ) Contribution of Cl − and non-Cl − conductance to urine-evoked currents in WT and TRPC2−/− mice. Current amplitude attributed to Cl − component (black bars) was calculated by subtracting the amplitude recorded using CsMSF from that using CsCl internal solution for both the WT and the TRPC2−/− VNO. The non-Cl − component (grey bars) was the current recorded using CsMSF internal solution. * P <0.05 and ** P <0.01 (pairwise t -test). All pairs marked with * have post hoc analysis of variance test, P <0.01. ext, external; int, internal. Full size image Intracellular Ca 2+ release activates CACC What was the Ca 2+ source to activate CACC in TRPC2−/− neurons? As TRPC2 was the only TRP family of ion channels identified in the VNO neurons [1] , [15] , [40] , we tested the possibility that Ca 2+ release from intracellular stores might trigger CACC activation. As the IP3 pathway had been implicated in VNO signalling [9] , we applied ruthenium red to block IP3-triggered intracellular Ca 2+ release in VNO neurons and examined the urine-induced current. We found that by blocking intracellular Ca 2+ release, urine-induced currents were reduced by 35.3±11.7% in WT VNO ( Fig. 4a,d ). We then used thapsigargin to deplete intracellular Ca 2+ stores and found that urine-induced currents were reduced by 51.5±8.8% ( Fig. 4a,d ). When we replaced intracellular Cl − with MSF − , the effects of ruthenium red or thapsigargin were eliminated ( Fig. 4c,d ). This observation suggested that the currents sensitive to these pharmacological reagents were mediated by Cl − . Moreover, urine-evoked responses in TRPC2−/− cells were completely blocked by ruthenium red or thapsigargin ( Fig. 4b,d ). Therefore, we concluded that IP3-mediated Ca 2+ release from intracellular stores were able to mediate the activation of the Cl − currents in WT and TRPC2−/− VNOs. In TRPC2−/− mice, the CACC current was activated through this pathway only. 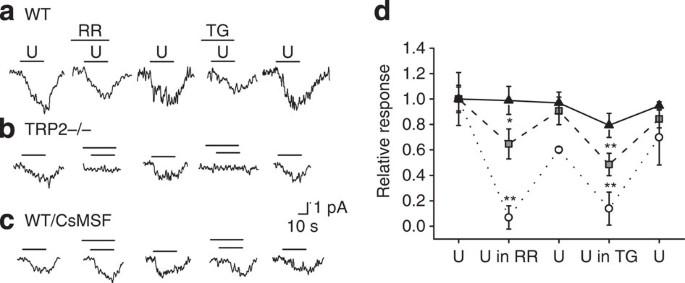Figure 4: Cl−conductance is dependent on intracellular release of Ca2+. (a–c) Sample traces of whole-cell current in VNO neurons from WT (a), TRPC2−/− (b) and WT with CsMSF internal solution (c) in response to first urine application (U), urine with 2 μM ruthenium red (RR), second urine application after washout (U), urine with 50 μM thapsigargin (TG) and third urine application after washout (U). (d) Relative response for each application in WT (n=9; grey squares), TRPC2−/− (n=7; white circles) and WT with CsMSF internal solution (n=6; black triangles). *P<0.05 and **P<0.01 for comparison with controls (pairwiset-test). All pairs marked with * havepost hocanalysis of variance test,P<0.01. Figure 4: Cl − conductance is dependent on intracellular release of Ca 2+ . ( a – c ) Sample traces of whole-cell current in VNO neurons from WT ( a ), TRPC2−/− ( b ) and WT with CsMSF internal solution ( c ) in response to first urine application (U), urine with 2 μM ruthenium red (RR), second urine application after washout (U), urine with 50 μM thapsigargin (TG) and third urine application after washout (U). ( d ) Relative response for each application in WT ( n =9; grey squares), TRPC2−/− ( n =7; white circles) and WT with CsMSF internal solution ( n =6; black triangles). * P <0.05 and ** P <0.01 for comparison with controls (pairwise t -test). All pairs marked with * have post hoc analysis of variance test, P <0.01. Full size image Requirement of CACC for VNO activation Is the Cl − current sufficient to drive the spiking activity of the VNO neurons? We recorded spiking activities of VNO neurons from WT and TRPC2−/− animals. To exclude the possibility that TRPC2 knockout might significantly alter the excitability of the neurons, we first examined the resting potential in WT and TRPC2−/− VNO neurons. We found that the resting potentials were indistinguishable among these neurons (WT: −51.07±0.64 mV, n =13; TRPC2−/−: −50.58±1.38 mV, n =12). We next performed extracellular recordings in order not to perturb the intracellular Cl − concentration. Application of urine elicited increases in spiking rates in WT and TRPC2−/− neurons alike, although the level of excitation in TRPC2−/− neurons was less than that in the WT neurons ( Fig. 5a–e , and Fig. 5f ). Treatment of the slices with niflumic acid or another Cl − channel-specific inhibitor, disodium 4-acetamido-4′-isothiocyanato-stilbene-2,2′-disulphonate (SITS), not only reduced the level of spontaneous activity of the VNO neurons but also blocked urine-induced increases in spiking rate ( Fig. 5a–e , and Fig. 5f ). The effects of niflumic acid and SITS could be reversed on washout ( Fig. 5a–e , and Fig. 5f ). Interestingly, we observed that when the Cl − channels were blocked, activation of the TRPC2 channels alone was not sufficient to excite the cells ( Fig. 5a,b,d ). This finding suggested that activation of CACC was required for VNO activation. 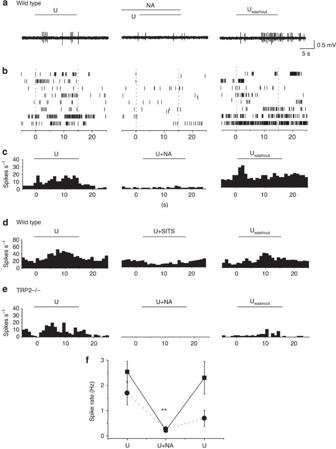Figure 5: Extracellular recording in VNO neuron. (a–c) Sample traces (a), raster plots (b) and peristimulus time histograms (c) of spiking activity in WT VNO neurons treated with urine alone (U), urine with 600 μM niflumic acid (NA),and second urine application after washout (Uwashout;n=8). (d) Peristimulus time histogram plots in urine alone (U), urine with 100 μM SITS and second urine treatment after washout (n=7). (e) Peristimulus time histogram plots in urine alone (U), urine with 600 μM niflumic acid (NA) and second urine treatment after washout (Uwashout) in TRP2−/− (n=7). (f) Spike rate change for neurons from WT (black squares) or TRP2−/− mice (black circles) in response to urine, urine with 600 μM niflumic acid (NA) and second urine treatment after washing out. **P<0.01 (post hocANOVA). Figure 5: Extracellular recording in VNO neuron. ( a – c ) Sample traces ( a ), raster plots ( b ) and peristimulus time histograms ( c ) of spiking activity in WT VNO neurons treated with urine alone (U), urine with 600 μM niflumic acid (NA),and second urine application after washout (U washout ; n =8). ( d ) Peristimulus time histogram plots in urine alone (U), urine with 100 μM SITS and second urine treatment after washout ( n =7). ( e ) Peristimulus time histogram plots in urine alone (U), urine with 600 μM niflumic acid (NA) and second urine treatment after washout (U washout ) in TRP2−/− ( n =7). ( f ) Spike rate change for neurons from WT (black squares) or TRP2−/− mice (black circles) in response to urine, urine with 600 μM niflumic acid (NA) and second urine treatment after washing out. ** P <0.01 ( post hoc ANOVA). Full size image In this study, we have investigated the role of CACCs in urine-evoked VNO activation and found that Cl − contributes to a significant portion of urine-evoked responses and is sufficient to drive spiking changes in WT and TRPC2−/− VNO neurons. We also demonstrated that CACC currents were able to mediate pheromone activation independently of TRPC2. In mice, olfactory cues are recognized by both the MOE and the VNO. The two sensory organs seem to have evolved independently using different sets of chemosensory receptors [1] , [2] , [3] , [5] , [6] , [7] and distinct signal transduction machineries [13] , [14] , [15] , [19] , [20] , [43] , [44] , [45] . Our study of the contribution of Cl − currents in VNO signalling further distinguished the two systems. The activation of the CACCs in the MOE is secondary to the cyclic-nucleotide-gated (CNG) channel. Ca 2+ entry through the CNG channel is required for the activation of the Cl − conductance [46] , [47] . Genetically, knockout of the CNG channel essentially abolishes odour-evoked current and renders the mice anosmic [48] . Our data show that the activation of the Cl − conductance in the VNO seems independent of the activation of the TRPC2 channel. In WT mice, ∼ 70% of the urine-evoked current is carried by Cl − under normal physiological conditions. TRPC2 carries ∼ 30% of the inward current, but Ca 2+ entry through TRPC2 is likely to further activate the CACC currents. Currents recorded from TRPC2−/− VNO are reduced by ∼ 50%, more than the currents carried by TRPC2. These observations indicate that Ca 2+ mobilization from intracellular stores and Ca 2+ entry through the TRPC2 channel act synergistically to activate the Cl − conductance. Nevertheless, without TRPC2, the CACC currents are able to excite the VNO neurons. When the Cl − channels are blocked, TRPC2 is insufficient to excite the cells. Thus, the CACCs seem to be necessary and sufficient to activate the VNO neurons. Our studies suggest a different view of CACC function in VNO activation from that of Yang and Delay [24] , who conclude that Cl − currents amplify inward currents mediated by other channels, as in the MOE. TRPC2−/− mice show striking phenotypes in sexual and aggressive behaviours [19] , [20] , [21] . The behavioural observations have also led to the notion that TRPC2 channel is the main contributor to VNO signalling. Our results show that the VNO neurons can be activated in TRPC2−/− mutants. These findings are consistent with electrophysiology studies from several other groups [11] , [22] , [49] and experiments showing remaining pheromone-elicited behaviours in TRPC2−/− mice [23] . Thus, the behavioural phenotypes observed in TRPC2−/− may not reflect the complete loss of VNO function. We note that, in TRPC2−/− mice, more than 50% of the basal layer of VNO neurons, which express the V2R family of vomeronasal receptors and the G o protein, are lost [19] (our unpublished observations). Thus, an alternative explanation of the behavioural phenotype in the TRPC2−/− mice is the combination of reduced VNO activation and selective loss of the basal layer of neurons. Animals Urine-evoked responses were obtained from 2- to 6-month-old male and female mice of C57BL/6J and TRPC2−/− [20] . The TRPC2 strain was backcrossed to C57/BL6J for at least three generations. Approximately equal numbers of male and female mice were used in the recordings. Urine was collected and stored at −20 °C as described previously [29] , [30] . For each experiment, urine samples were pooled from at least three male and three female mice. Animals were maintained in the Lab Animal Service Facility of Stowers Institute at 12:12 light cycle and provided with food and water ad libitum . Experimental protocols were approved by the Institutional Animal Care and Use Committee at Stowers Institute and in compliance with the National Institutes of Health (NIH) Guide for Care and Use of Animals. Electrophysiology Mice were killed by rapid cervical dislocation following CO 2 asphyxiation. Dissection of VNO tissue was performed in chilled mouse artificial cerebrospinal fluid (mACSF) aerated with 95% O 2 /5% CO 2. VNO was embedded in a gel composed of 4% low-melting-point agarose prepared in mACSF. Once the gel solidified, the tissue block was mounted on a specimen holder and secured onto the VF-300 microtome sectioning system (Precisionary Instruments). The VNO tissue was sectioned into 200 μm slices, which were then transferred to mACSF solution continuously aerated with 95% O 2 /5% CO 2 at room temperature. The composition of mACSF was (in mM): NaCl 125, KCl 2.5, CaCl 2 2, MgCl 2 1, NaHCO 3 25, Na 2 HPO 4 1.25 AND glucose (dextrose) 10. For external Cl − substitution experiments, NaCl was substituted with sodium gluconate. Patch clamp recording pipettes with resistance of 4–8 MΩ were fabricated using P-2000 micropipette puller (Sutter Instrument). A VNO slice was placed in a recording chamber continuously superfused with oxygenated mACSF. All recordings were performed using the Olympus BX50WI microscope equipped with a Rolera-XR camera (QImaging). A ×40 objective lens (NA 0.8) was used to guide patch pipette to individual neurons. Whole-cell recording was conducted using Multiclamp 700A amplifier (Molecular Devices), with 10 kHz sampling rate and low-pass filtered at 100 Hz for voltage clamp experiments and 1 kHz for current clamp recordings. The plotted current traces were low-pass filtered again at 20 Hz. For voltage clamp experiments, membrane potential was held at −60 mV, unless otherwise indicated. Current injection experiments were conducted under current clamp mode in whole-cell configuration. Current was clamped at I =0 at rest to maintain the original resting potential for the cell. Membrane potential was examined before and after current injection. The cells maintained resting potentials following the current injection. The following current injection protocols were applied. Five sweeps were made with 1 pA increment from 0 to 4 pA, followed by five sweeps with 3 pA increment from 5 to 17 pA and five sweeps with 5 pA increment from 15 to 35 pA. Changes in spike frequency were calculated by subtracting the spontaneous spike rate from those during current injection. Unless otherwise indicated, the pipette was filled with intracellular solution containing (in mM): CsCl 130, MgCl 2 2, CsOH 10, EGTA 1, HEPES 10, ATP 5 and GTP 0.3 in pH 7.2. Free Ca 2+ concentration in the recording solutions was estimated to be 5.55 nM (1 mM EGTA) according to McGuigan et al . [31] For internal Cl − substitution experiments, CsCl was substituted with caesium methanesulfonate. Urine from mature male and female mice was mixed at 1:1 ratio and diluted to 1:100 in mACSF for stimulation of the VNO slices. Urine was delivered for 15 sec using a pressurized perfusion system (ALA-VM8, ALA Scientific Instruments). The tip of the perfusion head is placed ∼ 500 μm away from the slice. The time delay of the stimulus was measured using a solution containing fluorescein. It took ∼ 300 ms from the start of the delivery for the dye signal to reach plateau value. The 15-sec delivery time mimicked the duration of a typical urogenital investigation episode for the mouse. For inhibitor experiments, VNO slice was incubated in mACSF containing 600 μM niflumic acid or 100 μM SITS for 2 min before stimulation. For extracellular recordings, pipettes with tip size around 1 μm and 1–3 MΩ resistance were fabricated and filled with mACSF. Recordings were performed in a loose patch configuration. A loose seal (80–100 MΩ resistance) was formed by applying gentle suction when the electrode tip was in contact with a cell. Signals were band filtered between 300 Hz and 3 kHz. How to cite this article: Kim, S. et al . Requirement of calcium-activated chloride channels in the activation of mouse vomeronasal neurons. Nat. Commun. 2:365 doi: 10.1038/ncomms1368 (2011).